C-SuFEx linkage of sulfonimidoyl fluorides and organotrifluoroborates Sulfur(VI) fluoride exchange, a new type of linkage reaction, has excellent potential for application in functional molecule linkage to prepare pharmaceuticals, biomolecules, and polymers. Herein, a C-SuFEx reaction is established to achieve fast (in minutes) linkage between sulfonimidoyl fluorides and aryl/alkyl organotrifluoroborates. Potassium organotrifluoroborates are instantaneously activated via a substoichiometric amount of trimethylsilyl triflate to afford organodifluoroboranes, releasing BF 3 as an activating reagent in situ. This sulfur(VI) fluoride exchange technique is capable of forming S(VI)-C(alkyl), S(VI)-C(alkenyl) and S(VI)-C(aryl) bonds, demonstrating its broad scope. Natural products and pharmaceuticals with sensitive functional groups, such as valdecoxib, celecoxib and diacetonefructose, are compatible with this protocol, allowing the formation of diverse sulfoximines. Since the concept of sulfur(VI) fluoride exchange (SuFEx) was first developed by Sharpless and coworkers in 2014 [1] , this efficient metal-free reaction has been widely applied in the formation of molecular linkages [2] , [3] , [4] , [5] , [6] in the fields of pharmaceuticals [7] , [8] , chemical biology [9] , and materials chemistry [10] , [11] , [12] . Sulfonimidoyl fluoride is a nitrogen isostere of sulfonyl fluoride possessing an adjustable handle for reactivity tuning and functional enhancement (Fig. 1A ) [13] , [14] , [15] . Sulfonimidoyl fluorides have been applied to form S(VI)-O [11] , [12] , [16] and S(VI)-N [7] , [17] , [18] linkages with phenols and amines as coupling partners, aiming to generate molecular connections for rapid and efficient target-based functional discovery (Fig. 1B ) [19] , [20] , [21] , [22] . However, the C-SuFEx [SuFEx for S(VI)-C bond formation] of sulfonimidoyl fluorides is limited to coupling with TMSCF 3 [23] , [24] and highly active organometallic reagents such as Grignard and lithium reagents [17] , [25] . It is imperative to establish a C-SuFEx technique that can be applied with a stable, mild and compatible partner. Effort has been made in our group to apply the C-SuFEx technique to alkynes via an intramolecular hydride transfer process [26] and to unactivated alkenes via an intermolecular hydride transfer process [27] , which requires a stoichiometric activating reagent for S(VI)-C bond construction [28] . Potassium organotrifluoroborates possess exceptional stabilities toward air and moisture [29] , [30] , [31] , [32] , [33] , [34] , [35] , and the electronegativity of potassium (0.8), which differs from those of fluorine (4.0) and oxygen (3.4), serves as a mediator via electrostatic attraction. Subsequently, a silicon-based Lewis acid has been applied to achieve a C-SuFEx linkage reaction via the interactions of Si···F (BDE = 135 kcal/mol) with potassium organotrifluoroborates via propagation steps involving tricoordinate/tetracoordinate boron species. Herein, we report the application of C-SuFEx to link sulfonimidoyl fluorides and aryl/alkyl organotrifluoroborates via the electrostatic attraction of potassium cation with F and O prompting silicon-based Lewis acid to activate S(VI)-F bonds (Fig. 1C ). The results of DFT theoretical calculations demonstrated that a lower Si-X (X = OTf, OMs, OAc, and Br) heterojunction bond energy for silicon-based Lewis acids and weak binding between RBF 2 and KX are the keys to the success of the propagation steps. Fig. 1: SuFEx chemistry and sulfoximines. a SuFEx linker, ( b ) bioactive sulfoximines, and ( c ) this work: the construction of diverse S(VI)-C bonds. Full size image 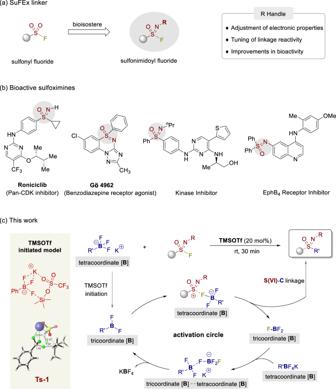Fig. 1: SuFEx chemistry and sulfoximines. aSuFEx linker, (b) bioactive sulfoximines, and (c) this work: the construction of diverse S(VI)-C bonds. We commenced the C-SuFEx linkage reaction of sulfonimidoyl fluoride 1a and phenyltrifluoroborate 2a with the assistance of an initiator, and disappointingly, the metal-based Lewis acids failed to generate the corresponding product (Table 1 , entry 1). Silicon-based Lewis acids were then tested due to the strong bonding energy between fluorine and silicon; fortunately, the desired sulfoximine product 3a was detected in less than 10% yield in the presence of TMSCl, TMSBr and TMSOAc (entries 2–4). Unexpectedly, the substoichiometric amount of TMSOTf and TBSOTf delivered desired product 3a in favorable yields (entries 5-6). However, a moderate yield was achieved by employing the Brønsted acid triflic acid as the initiator (entry 7). N -Tosyl and N -benzoxyl sulfonimidoyl fluorides failed to afford the corresponding C-SuFEx product 3 , and it is possible that electron-withdrawing groups are not conducive to stabilizing the sulfonimidoyl cation intermediate (entries 8-9). Further evaluation of the reaction solvents revealed that CH 3 CN was the optimal solvent for the current C(Ar)-SuFEx linkage reaction (entries 10-11). When the ratio of 1a to 2a was tested, product 3a was obtained in an almost quantitative yield with a 1.5:1 ratio (entry 12). Reducing the amount of TMSOTf at room temperature was not beneficial for the linkage (entries 13-14). However, raising the temperature slightly to 40 °C compensated for the impact of the lower quantity of Lewis acid on the C-SuFEx linkage efficiency, affording the sulfoximine in excellent yield (entry 15). It was found that cations of trifluoroborates other than potassium cation can still be compatible with the linkage (entries 16-18). Table 1 Conditions optimization a Full size table Subsequently, the linkage of sulfonimidoyl fluorides and organotrifluoroborates 2 was investigated comprehensively for a diverse sulfoximine library (Fig. 2 ). Substitution at the ortho- , meta- , and para- positions of the aromatic ring in potassium aryltrifluoroborate salts with electron-poor or electron-rich functional groups allowed formation of the target sulfoximine products ( 3b - 3h ) in good yields. The presence of steric hindrance on the substrate barely affected the linkage efficiency ( 3 h ). Conjugated aromatic ring systems, such as biphenyl, naphthalene, phenanthrene and pyrene, were well tolerated ( 3i - 3l ), especially for potassium (4-biphenyl)trifluoroborate, affording the product in a nearly quantitative yield. The linkage reaction was also efficient for potassium heteroaryltrifluoroborate salts with thienyl-, benzofuryl-, dibenzofuran-, and indolyl-derived substrates ( 3m - 3r ). The structure of 3 m was further confirmed via X-ray diffraction analysis (CCDC: 2240513). Notably, this strategy enabled the conversion of alkenyl and allyl potassium trifluoroborate salts as SuFEx partners ( 3 s and 3t ). To further expand the library of functionalized sulfoximines, various types of sulfonimidoyl fluorides were evaluated. In addition to ortho- , meta- , and para- substituted aryl sulfonimidoyl fluorides ( 3u - 3aa ), substrates containing conjugated aromatic rings ( 3ab - 3ad ) and heterocycles ( 3ae, 3af and 3ag ) proved to be competent linkage partners. The linkage of N -Et-, N - i Pr-, N - t Bu-, N -Bn- and N -Ph-substituted sulfonimidoyl fluorides proceeded smoothly, affording the desired sulfoximines ( 3ah-3al ). To our delight, alkyl and alkenyl sulfonimidoyl fluorides participated in the current C-SuFEx linkage with potassium trifluoroborate salts to generate the products in excellent yields ( 3am - 3ao ). Fig. 2: Substrate scope a . The C-SuFEx linkage reaction of sulfonimidoyl fluorides and potassium trifluoroborate salts. a Reaction conditions: 1a (0.6 mmol), 2a (0.4 mmol), TMSOTf (20 mol%), CH 3 CN (2 mL), N 2 , rt to 40 °C, 30 min; b TMSOTf (50 mol%), rt, air, 30 min; c TMSOTf (30 mol%). Full size image To further highlight the applicability of the current C-SuFEx linkage reaction, naturally occurring products and pharmaceuticals with sensitive functional groups and multiple heteroatoms were investigated (Fig. 3 ). The nonsteroidal anti-inflammatory drug valdecoxib allowed linkage with a benzothiophene and a naturally occurring estrone in good to excellent yields ( 3ap and 3aq ). The naturally occurring products coumarin and estrone could be linked efficiently via the current strategy ( 3ar ). The C-SuFEx linkage of the highly selective COX-2 inhibitor celecoxib and the hypolipidemic drug clofibrate was readily achieved using this methodology ( 3as ). Diacetonefructose containing multiple heteroatoms was amenable to the TMSOTf-catalyzed linkage as well ( 3at ). Additionally, the successful assembly of the anti-inflammatory drug flurbiprofen and the analgesic drug carprofen demonstrated the application value and prospects of this method for drug molecule linkage ( 3au ). Fig. 3: The linkage of functional molecules a . a Reaction conditions: 1a (0.6 mmol), 2a (0.4 mmol), TMSOTf (20 mol%), CH 3 CN (2 mL), N 2 , rt to 40 °C, 30 min. b TMSOTf (30 mol%). c TMSOTf (50 mol%), rt, air. Full size image To identify the mechanism of the TMSOTf-initiated linkage, the competition experiments of substituted sulfonimidoyl fluorides with different electron effects were conducted (Fig. 4 ). 4-OMe-substituted sulfonimidoyl fluoride afforded dramatically a higher yield compared to 4-CF 3 -substituted sulfonimidoyl fluoride for the corresponding products, demonstrating that electron-rich sulfonimidoyl fluorides display a faster rate than the electron-poor sulfonimidoyl fluorides. Subsequently, 19 F NMR studies were conducted (Fig. 5a ). When 20 mol% TMSOTf was added to 1a and 2a , TMSF was generated in the reaction systems, demonstrating the activation from TMSOTf on both substrates 1a and 2a . Moreover, the chemical shift of 1a shifted toward the high field region (Fig. 5a, I vs . VI), and new peaks appeared in the spectrum of 2a (−152.04 and −152.09 ppm) with a peak area ratio of 1:4 (Fig. 5a , VII). When one equivalent of TMSOTf was added to substrate 2a , the peak attributed to 2a (−143.59 ppm) and the abovementioned new peaks (−152.04 and −152.09 ppm) disappeared (Fig. 5a , VIII), but a peak attributed to PhBF 2 (−120.83 ppm) was observed. These results suggest that the new peaks may be attributed to a boron fluoride compound formed by PhBF 2 and unreacted 2a . During the model reaction, the fluorine signal of 1a did not change, indicating that TMSOTf interacted with 2a in the linkage reaction first. At the same time, a signal attributed to KBF 4 was observed in the spectrum (Fig. 5a , IX). Fig. 4: Competition experiments. Substituted sulfonimidoyl fluorides with different electron effects. Full size image Fig. 5: Mechanistic studies. a 19 F NMR studies in CD 3 CN. b Density functional theory (DFT) calculation: the energy profiles were calculated at 298.15 K at the level of M06-2X/6-311 G(d,p) SMD=acetonitrile. c Bond heterolysis energies of Si-X (X = O, Br) and binding energies of PhBF 2 with KX. Full size image Based on DFT theoretical calculations and verification (Fig. 5b ), an energy barrier of 10.2 kcal/mol is required to obtain Int-a when TMSOTf is applied for the activation of substrate 1a , and then the intermediate Int-b is obtained via the transition state TS-a . When TMSOTf interacts with substrate 2a , the energy decreases to allow formation of Int-1 , generating Int-2 from TS-1 , which is associated with an energy barrier of −24.7 kcal/mol. These results demonstrate that TMSOTf interacts with substrate 2a preferentially in the reaction. During the activation process, the B-F bond length of 2a is elongated from 1.44 Å ( Int-1 ) to 1.53 Å ( TS-1 ), resulting in the release of PhBF 2 , TMSF, and KOTf. Subsequently, PhBF 2 activates the S-F bond in 1a . The S(VI)-F bond length is extended from 1.67 Å ( Int-3 ) to 1.85 Å ( TS-2 ), resulting in the rapid release of the sulfonimidoyl cation ( Int-4 ) by overcoming an energy barrier of 2.3 kcal/mol. Target product 3a was obtained via phenyl migration, while BF 3 was dissociated with an energy barrier of −29.1 kcal/mol. During the activation process of BF 3 , BF 3 may activate either substrate 1a or 2a , and the DFT calculations show that BF 3 tends to activate phenylboron trifluoride potassium salt 2a (with an energy barrier of −6.8 kcal/mol) to afford Int-5 , while the interaction between sulfonimidoyl fluorides and BF 3 is associated with an energy barrier of 4.1 kcal/mol. Removal of the fluoride anion of 2a was achieved under the activation of BF 3 to form Int-6 , releasing KBF 4 and highly active PhBF 2 , thus initiating the next activation cycle. To further demonstrate the uniqueness of TMSOTf, different types of silicon-based Lewis acids were selected for control experiments (Fig. 5c ). The yield of this linkage reaction was optimal with TMSOTf, and a slight decrease in the yield was observed when TMSOMs was used. No target product 3a was generated with TMSOAc and TMSBr. A calculation of the reaction energy barriers showed that TMSOTf possessed a lower Si-O bond heterojunction energy and a lower energy barrier for different Lewis acids with potassium phenyltrifluoroborate 2a (Supplementary Fig. 9 ). The potassium salt, generated by the reaction of the Lewis acid with 2a , was not easily dissociated from PhBF 2 , thereby hindering the reaction. The binding energies of different potassium salts and PhBF 2 were calculated, and the binding energy of KOAc was the highest (25.4 kcal/mol). Although the Si-Br bond heterolysis energy of TMSBr was moderate (50.4 kcal/mol vs. 70.5 kcal/mol), the energy barrier of the reaction of TMSBr with potassium phenyltrifluoroborate 2a was higher (33.1 kcal/mol vs . 25.3 kcal/mol). Based on these experimental results, a reaction mechanism was predicted, as shown in Fig. 6 . 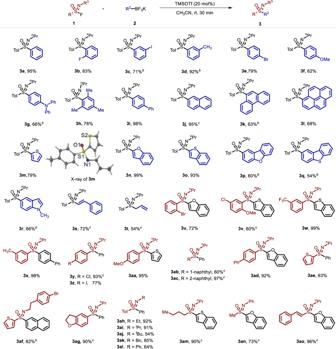Fig. 2: Substrate scopea. The C-SuFEx linkage reaction of sulfonimidoyl fluorides and potassium trifluoroborate salts.aReaction conditions:1a(0.6 mmol),2a(0.4 mmol), TMSOTf (20 mol%), CH3CN (2 mL), N2, rt to 40 °C, 30 min;bTMSOTf (50 mol%), rt, air, 30 min;cTMSOTf (30 mol%). Potassium phenyltrifluoroborate 2a is first activated by TMSOTf to generate PhBF 2 , releasing TMSF and KOTf. The S(VI)-F bond of sulfonimide fluoride 1a is activated by PhBF 2 to obtain sulfonimide thiocation pair Int-4 via Int-3 . The aryl group migration afforded target product 3a , releasing BF 3 , which is activated with 2a to regenerate phenylboron difluoride and KBF 4 to complete the activation process. Fig. 6: The key catalytic cycle. The catalytic cycle that including initiation, activation and aryl migration processes. Full size image In conclusion, a TMSOTf-initiated C-SuFEx reaction of sulfonimidoyl fluorides and potassium organotrifluoroborates was established to synthesize a range of sulfoximines. A substoichiometric amount of TMSOTf activated stable and commercially available potassium organotrifluoroborates to release organodifluoroboranes, which interacted with sulfonimidoyl fluorides to generate BF 3 in situ as an activating reagent to achieve efficient linkage. A range of naturally occurring molecules and pharmaceuticals with multiple heteroatoms and sensitive functional groups were highly compatible with this linkage reaction, furnishing functional sulfoximines. Mechanistic studies and DFT calculations further revealed that trimethylsilyl triflate activated potassium organotrifluoroborates first and released organodifluoroboranes in situ. A lower Si-X (X = OTf, OMs, OAc, and Br) bond heterojunction energy of silicon-based Lewis acid and a weak binding of RBF 2 with KX are the keys to the success of this C-SuFEx process. Further application of C-SuFEx of sulfonimidoyl fluorides is in progress in our laboratory. General reaction procedure Under nitrogen atmosphere, dry CH 3 CN (2 mL, 0.2 M) was added to a 10 mL oven-dried Schlenk tube, which was equipped with sulfonimidoyl fluoride 1 (0.60 mmol), potassium organotrifluoroborate salt 2 (0.40 mmol) and a stirring bar. TMSOTf (0.08 mmol) was dropwise added via the microsyringe at room temperature. 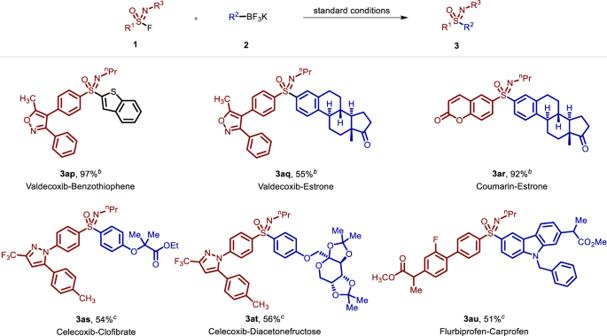Fig. 3: The linkage of functional moleculesa. aReaction conditions:1a(0.6 mmol),2a(0.4 mmol), TMSOTf (20 mol%), CH3CN (2 mL), N2, rt to 40 °C, 30 min.bTMSOTf (30 mol%).cTMSOTf (50 mol%), rt, air. Then the reaction mixture was stirred at 40 o C for 30 min and quenched with saturated aqueous solution of sodium carbonate. 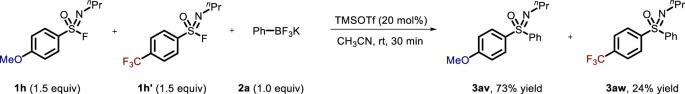Fig. 4: Competition experiments. Substituted sulfonimidoyl fluorides with different electron effects. After the extraction of DCM for three times, the organic phase was washed with brine and dried over anhydrous Na 2 SO 4 . 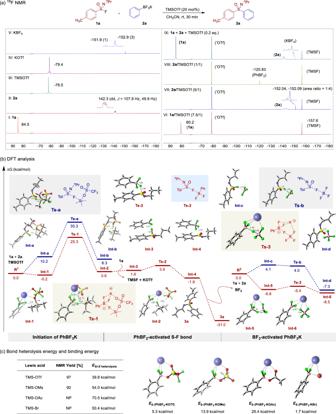Fig. 5: Mechanistic studies. a19F NMR studies in CD3CN.bDensity functional theory (DFT) calculation: the energy profiles were calculated at 298.15 K at the level of M06-2X/6-311 G(d,p) SMD=acetonitrile.cBond heterolysis energies of Si-X (X = O, Br) and binding energies of PhBF2with KX. 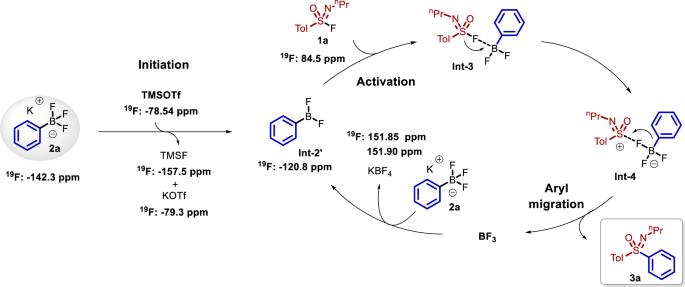Fig. 6: The key catalytic cycle. The catalytic cycle that including initiation, activation and aryl migration processes. The solvent was evaporated under reduced pressure, and the residue was purified by column chromatography to yield the corresponding sulfoximine product 3 .